Information on quantum states pervades the visible spectrum of the ubiquitous Au144(SR)60gold nanocluster Absorption spectra of very small metal clusters exhibit individual peaks that reflect the discreteness of their localized electronic states. With increasing size, these states develop into bands and the discrete absorption peaks give way to smooth spectra with, at most, a broad localized surface-plasmon resonance band. The widely accepted view over the last decades has been that clusters of more than a few dozen atoms are large enough to have necessarily smooth spectra. Here we show through theory and experiment that for the ubiquitous thiolate cluster compound Au 144 (SR) 60 this view has to be revised: clearly visible individual peaks pervade the full near-IR, VIS and near-UV ranges of low-temperature spectra, conveying information on quantum states in the cluster. The peaks develop well reproducibly with decreasing temperature, thereby highlighting the importance of temperature effects. Calculations using time-dependent density-functional theory indicate the contributions of different parts of the cluster–ligand compound to the spectra. Colourful and iridescent materials, endowed with tremendous aesthetic and practical characteristics by noble-metal clusters, were prized already in antiquity. Recently, these clusters have taken the centre stage as critical agents in emerging technologies—in optics; in electronics; in diagnostic; and in therapeutic medicine [1] , [2] , [3] , [4] , [5] , [6] . Gold and gold-alloy clusters can act as intense pigments of high durability in spectral ranges perfectly suited to human colour-vision (VIS) owing to the characteristic Mie Bands (or localized surface-plasmon resonances, LSPR) that predominate in that region [7] , [8] . The—still open—practical question concerning the ultimate limits of miniaturization of plasmonic clusters requires a fundamental physical understanding including the quantum nature of the clusters [9] , [10] , [11] . The high stability and the size of the ubiquitous monolayer-protected 144-atom noble-metal cluster compound Au 144 (SR) 60 confer a special role as a very suitable prototypical system. Its thiolate (RS-) groups include both a sulphur (S) atom and a rest (R) group, typically organic. The size of Au 144 (SR) 60 is in the transition range critical for a fundamental understanding of the metal clusters’ physics. Here, the quantum information in the spectra emerges but no strong LSPR covers the details of the spectra yet. Moreover, high stability leads to high reproducibility of experiments. Many groups have studied this compound [12] , [13] , [14] , [15] , [16] with varying thiolate ligands and, more recently, with noble-metal compositions varying between pure gold and different Au–Ag [17] and Au–Cu [18] alloys. These clusters are notable for their compact symmetrical structure, well-defined electrical capacitance, and optical and electronic properties. Their structure has been experimentally confirmed [19] , [20] . The designation has varied over time. Earlier work, before the advent of complete compositional characterization, referred to clusters of ‘~150 Au atoms’; other cited numbers were 140, 146 and 147. The core mass of 29 kDa has also often been used to characterize the compound [16] . Apart from the fundamental scientific interest, the selected cluster has been commercially available since many years (‘PeptideGold’ [3] ) and in continuous use in biological and medical investigations over the past decade: bioconjugation chemistry [21] , protein tagging [3] , biomolecule labelling [4] , inhibition of HIV fusion [5] and growth inhibition of bacteria [6] are but a few of its applications. Small noble-metal clusters are finite systems and necessarily have discrete electronic energy levels. With increasing size, these discrete levels start to develop into the bands that characterize the bulk metals. The optical response of the clusters reflects the nature of the electronic states. Spectroscopic measurements that characterize the features of the absorption spectra thus provide information on the quantum nature of the clusters, on their electronic states, and on the ‘quantum size effects’ that influence them. In line with the change of the electronic states, the spectra show a transition from quasi-molecular spectra with a number of distinct peaks (a few dozen atoms) to smooth large-cluster spectra without distinct peaks—except, in many cases, for a smooth, broad LSPR band. However, it must be emphasized that the emergence of the LSPR is a phenomenon that is clearly distinct from the transition from the discrete to the smooth spectrum. The correspondence between the discrete electronic levels or bands in the cluster with the distinct peaks in the spectra is not trivial. As optical measurements necessarily involve electronic excitations, the dynamics of the excited states plays a substantial role; their lifetime in the interacting many-electron system introduces a broadening of the transitions even if lattice vibrations are neglected [22] , [23] . In addition, thermal lattice vibrations increase the broadening. Moreover, even for zero temperature, the zero-point motion has a non-negligible influence on optical spectra [24] . Consequently, the question whether the spectra of a given cluster compound such as the Au 144 (SR) 60 will show individual peaks is far from trivial even at very low temperature. The different previous measurements of optical absorption spectra of Au 144 (SR) 60 (for cases of all-Au and R=aliphatic) show a high degree of agreement in the range between 0.5 and 4.5 eV: weak absorption features in the infrared (0.4–1.5 eV) yield to a strong rise, centred near 1.6 eV, generally attributed to the onset of interband transitions from the 5d electrons. A minor peak at ~1.8 eV and two broad maxima that were not further resolved previously (~2.3 and 3.2 eV) dominate the visible region. Minor undulations appear over the spectrum (or step-like features, in the differential spectra) that are well reproduced but of unknown origin [15] , [16] . Little is known about the exact way the transition from spectra with distinct peaks to smooth spectra takes place, about even the precise size range and the factors that influence it. The prevalent view in recent decades has been that noble-metal clusters of intermediate size—that is, those with more than a few dozen but fewer than ~10 3 metal atoms—necessarily have featureless optical absorption spectra of low information content in the near-IR, VIS and near-UV regions. At most, one expects a broad, smooth LSPR feature [25] , [26] . High information content is expected only in the mid-IR region [27] . This view is stated in the oldest references [27] , [28] , [29] that are 25 years old, but also, for example, in very recent reviews [30] , [31] . The latest restatement of this point of view is found in the very recent work of Malola et al. [26] that apparently reports the first time-dependent density-functional theory (TD-DFT) spectra in the visible region of the Au 144 cluster. The article specifically states that ‘[Au 102 and Au 144 clusters] have rather featureless spectra,’ in agreement with the results presented therein. Herein we demonstrate that, in contradistinction to the commonly held view, the optical absorption of the most widely applied gold cluster, the (thiolate) monolayer-protected Au 144 compound (~1.6-nm-core diameter) exhibits a rich spectrum of bands that are individually visible over the entire near-IR, VIS and near-UV regions (1.0–4.0 eV), demonstrating high information content related to the quantum size effects, which distinguish the nanoparticles from the bulk materials [27] . The results were obtained owing to low-temperature measurements on ultra-homogeneous samples [32] and realistic quantum-theoretical [33] simulation (~2,500 active electrons). Our results call for fundamental re-evaluation of the perceived limits to ‘quantum information content’ of spectra in the crucial size range between 100 and 300 metal atoms, wherein the plasmonic response first emerges in the stable cluster materials actually employed in science and technology applications. Optical measurements The new experiment, shown in Figs 1 and 2 , reveals how sample cooling brings forth a clear and well-resolved multiple-band structure. The low-temperature measurement shows nine clearly distinct peaks in the main range between 1.8 and 4.5 eV. Two more peaks and a smaller feature are found in the low-energy region between 1.0 and 1.7 eV. Comparison of the room-temperature result and the low-temperature 77 K measurement shows clearly the development of the peak structure with temperature; thermal broadening obscures the intrinsic fine structure of the spectrum. This is even more clearly seen in the inset of Fig. 2 where we show the difference between the low temperature and the room-temperature measurements. The full series of measurements is shown in Supplementary Fig. 1 , demonstrating the gradual emergence of the individual peaks with decreasing temperature. The presentation in Fig. 2 is complemented by Supplementary Fig. 2 , showing the absorbance plotted against the wavelength. The rather general validity of these measurements for the Au 144 compounds is underlined by the comparison with measurements on Au 144 (SC 2 H 4 Ph) 60 —that is, with a different ligand rest group—shown in Supplementary Fig. 3 . Even though the lowest temperature was 177 K in this case, the incipient development of the individual peak structures is discernable. The main effects that obscure these individual peaks at room temperature are the thermal vibrations of the ‘lattice’, the possible switching between the multiple conformers of similar energies of the cluster–ligand system and the increase in inhomogeneity in the direct surroundings of the clusters. Therefore, in addition to the fabrication of ultra-homogeneous samples, a low-temperature measurement is indispensable for the detection of these features. 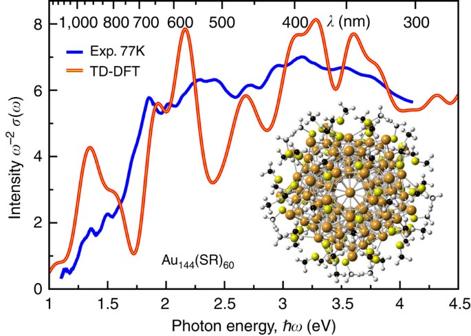Figure 1: Low-temperature measurement and TD-DFT calculation of the optical spectra of Au144(SR)60. In the calculation (red), R=CH3, while in the measurement (blue), R=C6H14. (The low sensitivity to different ligands is demonstrated in SupportingFig. 3.) Plotted is the optical absorption cross-section,σ(ω), frequency-weighted (ω−2) to match the optical-absorbance function,σ(λ), versus the optical frequency,ω, in electron volt (eV) units of the photon energy (ℏω). Figure 1: Low-temperature measurement and TD-DFT calculation of the optical spectra of Au 144 (SR) 60 . In the calculation (red), R=CH 3 , while in the measurement (blue), R=C 6 H 14 . (The low sensitivity to different ligands is demonstrated in Supporting Fig. 3 .) Plotted is the optical absorption cross-section, σ ( ω ), frequency-weighted ( ω −2 ) to match the optical-absorbance function, σ ( λ ), versus the optical frequency, ω , in electron volt (eV) units of the photon energy ( ℏ ω ). 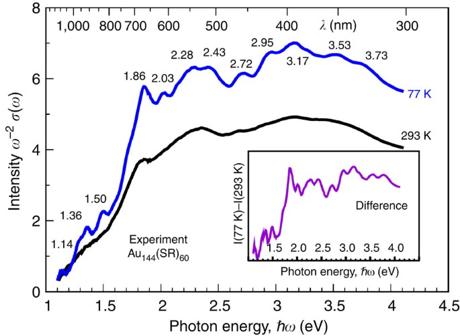Figure 2: Experimental absorption spectra of Au144(SR)60. R=C6H13, we show the spectra at room temperature 293 and at 77 K. The inset shows the difference between the room temperature and the low-temperature measurements. The complete series of spectra of intermediate temperatures is shown inSupplementary Fig. 1. Full size image Figure 2: Experimental absorption spectra of Au 144 (SR) 60 . R=C 6 H 13 , we show the spectra at room temperature 293 and at 77 K. The inset shows the difference between the room temperature and the low-temperature measurements. The complete series of spectra of intermediate temperatures is shown in Supplementary Fig. 1 . Full size image TD-DFT calculations The calculation of the clusters’ optical properties on the quantum level is cumbersome because of the large size of the system. TD-DFT provides a method to take into account the inherent excitation aspect; however, it is numerically very demanding. Many TD-DFT studies have considered only the noble-metal’s 6 s electrons explicitly, approximating the remaining ionic cores as a smooth charge background in the so-called jellium model, and describing the filled shell of the polarizable 5 d electrons by an appropriate dielectric function derived from the optical functions of the bulk material [34] , [35] . Consequently, these calculations cannot precisely describe the contributions from the 5d band and, in particular, not the strong quantization effects in the 5 d bands that alter the properties of the quantum-sized clusters with respect to the bulk metal. Precisely in Au clusters where the 5d band starts just 1.8 eV below the Fermi energy, these contributions become decisive. For instance, in Au nanorods, where the energy of the longitudinal LSPR depends essentially on the aspect ratio, even the character of the response can be changed by coupling or decoupling the resonance from the interband transitions by means of changes of the aspect ratio [36] , [37] . The calculation of the optical spectra of Au clusters must, therefore, explicitly consider the 5 d electrons. This is possible with TD-DFT using pseudopotentials. The resulting calculations are numerically demanding—about 2,500 electrons must be included explicitly as valence electrons—but enable the proper description of the bonding and interaction with the ligand shell. For the calculations, it is important to know the precise structure of the clusters and the ligand shell. For a number of Au clusters, structures have been determined experimentally using X-ray diffraction [38] . However, the total structure determination of the respective cluster compounds remains challenging. The ground-state electronic structure and the bonding with the ligands of the title compound have been investigated by Malola et al. [39] The structure model employed by these authors has subsequently been improved owing to recent experimental results that point to high-symmetry structures [19] . Recently, the generally accepted structure has been improved for the Au 144 (SR) 60 using STEM Electron Diffraction and high-resolution imaging along with ground-state calculations of static DFT [20] . The structure (see Fig. 1 ) comprises four concentric shells of atoms: the inner core consists of shells of 12+(30+12) Au atoms and has no coordination to ligands; the Grand Core (114 Au atoms) consists of the inner core plus 60 surface Au atoms, each singly coordinated to thiolate (RS-); the final (4th) shell is the protective layer comprising 30 staple-motif units (RS-Au(I)-SR)—that is, the ligands of this compound include themselves gold ad-atoms [20] , [38] , [40] , [41] . One would, therefore, generally expect a rather strong influence of the ligands, defined herein to include both the 30 Au(I) ad-atoms and the thiolate groups, on the optical spectra. At the onset of optical absorption—that is, in the region of the optical gap—TD-DFT has been used by Koivisto et al. [42] to calculate the optical spectrum in rather good agreement with experiment up to about 0.6 eV using transition-based calculations, employing the lower-symmetry model of previous work [39] . However, the visible and near-UV spectral regions have so far been out of reach for atomistic TD-DFT calculations of this cluster size because of the large number of transitions that need to be taken into account to converge the spectra up to the desired energy. The first calculation of the VIS range [26] has been published in late 2013. The influence of ligands on the electronic and optical properties has been studied for a number of smaller systems, see for example refs 43 , 44 , 45 , 46 . The spectra of ligand-coated Au 55 and Au 69 clusters have been calculated by Burgess et al. [47] who concluded that the coating reduces the features present in the spectra of the bare clusters. However, the ligands considered in their study do not contain staple-motif units. In the present study, we apply TD-DFT using pseudopotentials and the time-evolution formalism [48] to calculate the optical spectra in the visible and near-UV for the Au 144 (SCH 3 ) 60 cluster. In this approach, the time evolution of the system is calculated after an initial perturbation. The absorption spectrum is obtained from the time-dependent dipole moment. An illustration of the method is found in Supplementary Fig. 4 , a comparison with a transition-based calculation in Supplementary Fig. 5 . The approach has been successfully applied to investigate the size evolution of the optical response, describing both quantum-size effects and LSPR emergence of bare clusters of up to 263 Au and Ag atoms incorporating the sp conduction electrons and the filled d shell (~3,000) [33] , [36] , [49] . The advantage of the method is that no large number of empty states needs to be calculated, which allows us to converge the spectra up to at least 5.0 eV for the Au 144 (SCH 3 ) 60 cluster, thus covering the visible and near-UV spectral regions entirely. Calculated optical spectra The absorption spectra of the TD-DFT quantum calculation of the Au 144 (SR) 60 cluster are compared with the low-temperature measurement in Fig. 1 . The striking finding, coherently demonstrated by both theory and experiment, calls for comprehensive, in-depth revision of the current widely accepted understanding of the optical response of these gold nanoparticles: the spectrum is replete with peaks and other fine structure, all reproducible (see Supplementary Figs 1 and 3 ), in contrast to the prevailing view that expects featureless spectra of low information content in the visible and near-UV spectral regions. The TD-DFT calculation reproduces the overall shape of the experimental spectra, although the individual peaks are more pronounced in the calculation. A clear correspondence between the different peaks is evident, in particular for the steep onset and the first peak measured at 1.86 eV and the two double-peak features at 2.95 and 3.17 eV and 3.53 and 3.73 eV. The energy range between 2.0 and 2.6 eV shows the most notable difference; the three distinct peaks at 2.03, 2.28 and 2.43 eV in the measurement compare with only one peak, of higher intensity, in the calculation. In the low-energy part of the spectrum, the correspondence is likewise clear for the two peaks measured at 1.36 and 1.50 eV, although the intensity in the calculation is apparently overestimated, as well as for the small feature at 1.14 eV. The remaining discrepancies between experiment and calculation in Fig. 1 are attributable to a number of minor influences. First, the calculation represents the result for fixed atomic positions, thus automatically excluding the effect of lattice vibrations. Calculations of the influence of the lattice vibrations have been performed in the framework of DFT/TD-DFT for a number of smaller nanostructures [50] , [51] , [52] . However, for the size of the Au 144 (SR) 60 compound, these calculations are not practicable. In addition, the direct inclusion of the electron–phonon coupling in the framework of ab initio calculations [24] is unlikely to be practicable for the clusters of the size of interest here soon. It is clear from the gradual emergence of the peaks in the experiment that further temperature decrease will lead to peaks that are even more strongly pronounced, thus removing part of the disagreement with the calculation. This is particularly important at low energy where the intensity of the two small peaks at 1.36 and 1.50 eV, shown below to reflect the contribution of the ‘staples’ in the ligands, are overestimated in the calculation. An earlier report on the smaller Au 25 and Au 38 clusters [32] found that cooling causes an enormous increase in cross-section in the low-energy range (1.0–1.5 eV). Therefore, in addition to the emergence of the two peaks from the rather smooth spectrum at room temperature as demonstrated in our measurement (see Fig. 2 and in particular Supplementary Fig. 1 ), we expect a large further increase in the intensity of these peaks upon further cooling, leading to even better agreement between experiment and calculation. Second, omitted from the theory are the finite lifetimes of the excited electrons and holes that derive from the electron–electron interaction of the many-body system [22] . The necessarily finite duration (25-fs in our case) of the calculated time evolution of the electronic system introduces an energy-independent lifetime-like broadening of ~0.15 eV. However, the lifetime effects, which are largely neglected in the adiabatic approximations of the exchange-correlation functional [23] , increase with the transition energy. This means that the sharp onset and peak at 1.8 eV will experience less additional broadening than the peaks at higher energy, which will bring the calculated spectrum into even better agreement with the experiment. Moreover, although in gold clusters the choice of the exchange-correlation functional in the TD-DFT calculation is not expected to alter the results significantly (see Supplementary Fig. 6 ), the details of the spectra might still be influenced. The same is true for the spin–orbit interaction, which is neglected in practically all calculations, including ours. The spin–orbit interaction introduces energetic splittings of transitions. For the lowest non-forbidden line in the Au atom, the splitting is as large as 0.5 eV (ref. 53 ). The splitting is likewise important in, for example, monoatomic Au chains [54] . However, for more compact Au clusters, the effect tends to be quenched, although it remains visible in the spectrum of, for instance, the 20-atom Au tetrahedron [54] . Similarly, a splitting of ~0.25 eV was found for the lowest peaks in the spectrum of a 41-atom Ge nanocrystal [55] . Comparing with these results, the spectra of the Au 144 (SR) 60 compound are not expected to change drastically, although details may certainly be modified. It is, in particular, possible that the spin–orbit interaction would improve the agreement between experiment and calculation by redistributing and shifting the intensity of the strong peak at 2.15 eV in the calculation. Third, the medium dielectric effect is omitted, which may give rise to a small (red-) shift of the experimental spectra. Fourth, the thiolate ligands are simpler in the theory than those employed experimentally. Finally, despite every effort, the experimental samples may suffer from residual inhomogeneities (in cluster structure, charge-state, glass-induced disorder and so on) that will degrade the spectral resolution. In view of these differences, the agreement between theory and experiment is rather good and provides a reliable basis for the assignment of the peaks and the conclusions drawn in the present study. Contribution of core and ligands To determine the origin of the different features in the spectra, we compare in Fig. 3 the absorption cross-section of the different shell structures to that obtained for the complete cluster. Physically, the most meaningful comparison contrasts the full Au 144 (SCH 3 ) 60 cluster (red line) against the Grand Core (black line) because this reveals directly the overall influence of the ligands including the gold ad-atoms. One observes a strong increase in the absorption in the VIS because of the ligands, in particular in the range between 1.75 and 2.3 eV. However, the three peaks below 2 eV of the full spectrum are absent in the spectrum of the Grand Core, leading directly to the conclusion that the inclusion of the ligands (staples) is required to obtain a satisfactory description of this portion of the spectrum. This is further corroborated by the fact that similar pure-Au clusters give spectra that differ only very little, as shown in Fig. 4 : the 140-atom truncated octahedron and the 147-atom icosahedron, nearest in size to the Au 114 and Au 144 subsystems investigated herein, produce very similar spectra, especially below 3 eV. One finds a multiband spectrum, with weaker features compared with the Au 144 cluster, dispersed across the entire visible-near-UV ranges [33] , [49] . In particular, the gold character without LSPR is not changed; the difference with a silver cluster of the same size, which shows a strong plasmonic resonance, is much greater than the differences between the different Au clusters. 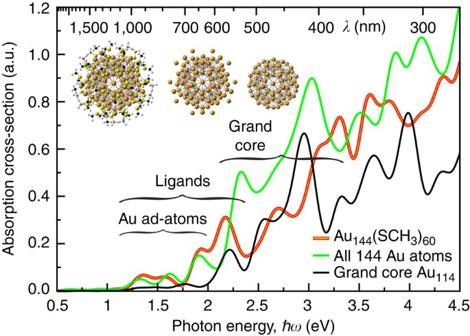Figure 3: Spectra of the full Au144(SR)60cluster and partial structures. The absorption cross-section of the full Au144(SR)60cluster, with R=CH3(left image), is compared with that of the Grand Core of 114 Au atoms (right), and to that of thead hocstructure consisting of all 144 Au atoms of the full cluster (middle image). The ligands are defined to include both the Au ad-atoms and the thiolate groups. Figure 3: Spectra of the full Au 144 (SR) 60 cluster and partial structures. The absorption cross-section of the full Au 144 (SR) 60 cluster, with R=CH 3 (left image), is compared with that of the Grand Core of 114 Au atoms (right), and to that of the ad hoc structure consisting of all 144 Au atoms of the full cluster (middle image). The ligands are defined to include both the Au ad-atoms and the thiolate groups. 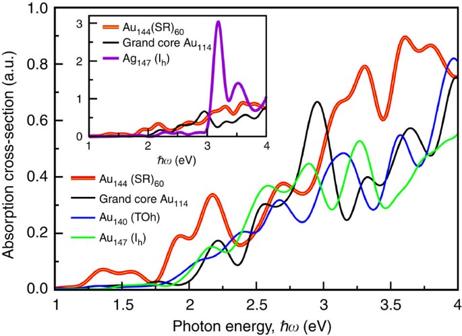Figure 4: Spectra of the thiolated Au144(SR)60compared with bare Au clusters. The absorption cross-section of the full thiolated Au144(SR)60cluster, R=CH3, is shown along with the spectra of the Grand Core Au114and the 140-atom truncated octahedron and the 147-atom icosahedron. Inset: comparison of the full cluster Au144(SCH3)60and the Grand Core Au114with the 147-atom silver icosahedron. Full size image Figure 4: Spectra of the thiolated Au 144 (SR) 60 compared with bare Au clusters. The absorption cross-section of the full thiolated Au 144 (SR) 60 cluster, R=CH 3 , is shown along with the spectra of the Grand Core Au 114 and the 140-atom truncated octahedron and the 147-atom icosahedron. Inset: comparison of the full cluster Au 144 (SCH 3 ) 60 and the Grand Core Au 114 with the 147-atom silver icosahedron. Full size image In order to further elucidate the origin of the three peaks below 2 eV, we compare with the spectra of the ad hoc all-Au structure that contains all the 144 gold atoms of the full cluster but from which all the other atoms have been removed. The resulting structure consists of the Grand Core and the Au ad-atoms from the ligands at their original positions in the staple units. The spectrum of this structure is almost identical to the spectrum of the full cluster up to 2 eV. Together with the absence of these structures in the spectrum of the Grand Core, this implies that the thiolate groups may be unnecessary to obtain a satisfactory description of this portion of the spectrum. By contrast, the peak at 2.2 eV corresponds evidently to the peak of the spectrum of the Grand Core, apart from the strong increase in the absorption in this range. This peak and the spectrum up to ~3 eV are very similar to the spectrum of the Grand Core. It is, therefore, safe to assume that this part of the spectrum mainly originates from the core structure. A comparison of the electronic density of states of the full Au 144 (SCH 3 ) 60 and the partial shell structures, shown in Fig. 5 , is likewise instructive. The most important finding is that the onset of the 5 d band at ~1.8 eV in the Au 144 (SCH 3 ) 60 is much less steep than for the various considered Au-only structures. We note that this cannot be explained by a simple addition of states belonging to the ligands because in the interval 1.6–2.5 eV the DOS of the full thiolated Au 144 (SCH 3 ) 60 cluster is in fact rather strongly reduced compared with the DOS of the Grand Core. In other words, the addition of the thiolates including the Au atoms in the staple motifs reduces the density of states there, which can only be the case if the ligands induce a strong modification of the electronic structure. This leads to the conclusion that the ligands interact rather strongly with the core structure. The effect is seen even more strongly in the comparison with the ad hoc all-Au structure, although in this case the influence of the semi-isolated Au ad-atoms cannot easily be evaluated. 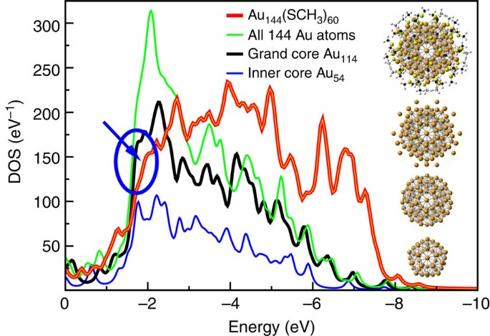Figure 5: Density of occupied states of the full and partial clusters. We show the DOS of the Kohn–Sham ground-state calculation for the full Au144(SR)60cluster, with R=CH3, compared with that of the Grand Core of 114 Au atoms and that of thead hocstructure of all 144 Au atoms. These are the structures for which the spectra are compared inFig. 3. In addition, we show the DOS of the Inner Core, Au54. The occupied states shown here belong mostly to thedband. The zero of the energy axis is the Fermi energy, a broadening of 0.1 eV is applied. Figure 5: Density of occupied states of the full and partial clusters. We show the DOS of the Kohn–Sham ground-state calculation for the full Au 144 (SR) 60 cluster, with R=CH 3 , compared with that of the Grand Core of 114 Au atoms and that of the ad hoc structure of all 144 Au atoms. These are the structures for which the spectra are compared in Fig. 3 . In addition, we show the DOS of the Inner Core, Au 54 . The occupied states shown here belong mostly to the d band. The zero of the energy axis is the Fermi energy, a broadening of 0.1 eV is applied. Full size image In order to investigate the interaction of the core with the ligands further, we check the simple possibility of adding the DOS of the different parts of the full cluster. In addition to the densities shown in Fig. 5 , we show in Fig. 6 the DOS of the ligand shell, including the Au ad-atoms, and of the shell of all non-Au atoms. Interestingly, the densities of states of the Grand Core Au 114 and of the ligand shell, as well as of the ad hoc all-Au cluster and of the remainder—that is, of the shell of all non-Au atoms—add up relatively precisely to the total density of states, except in the energy region between 1.5 and 2.5 eV, which shows once more that a strong interaction between the ligands and the core structure exists there. This is particularly interesting because the transition from the occupied states in this energy range just across the Fermi energy can contribute to the spectra in the range 1.75–2.5 eV which is, as shown in Fig. 1 , the region in which the absorption of the thiolated cluster is strongly increased compared with the Grand Core alone. 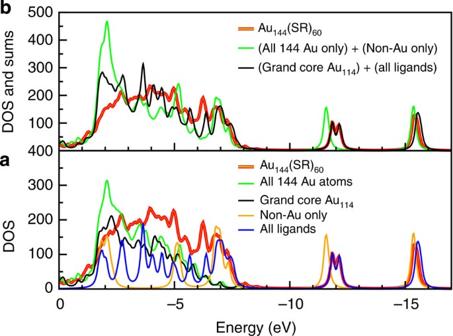Figure 6: Additivity of DOS of partial clusters. (a) Density of states of the full thiolated Au144(SR)60, R=CH3, and of the following partial structures: thead hocstructure of all gold atoms Au144, the Grand Core Au114, the shell of all non-Au atoms, as well as the shell of all ligands, including the Au atoms in the staple motifs. The zero of the energy axis is the Fermi energy, except for the latter twoad hocshell structures, which were shifted so as to agree with the lower part of the d-band-related broad contribution, between −6 and −8 eV. (b) Density of states of the full thiolated Au144(SR)60, R=CH3, compared with the sum of the densities of states as indicated. Figure 6: Additivity of DOS of partial clusters. ( a ) Density of states of the full thiolated Au 144 (SR) 60 , R=CH 3 , and of the following partial structures: the ad hoc structure of all gold atoms Au 144 , the Grand Core Au 114 , the shell of all non-Au atoms, as well as the shell of all ligands, including the Au atoms in the staple motifs. The zero of the energy axis is the Fermi energy, except for the latter two ad hoc shell structures, which were shifted so as to agree with the lower part of the d-band-related broad contribution, between −6 and −8 eV. ( b ) Density of states of the full thiolated Au 144 (SR) 60 , R=CH 3 , compared with the sum of the densities of states as indicated. Full size image Combining state-of-the-art low-temperature absorption measurements on ultra-homogeneous samples and realistic quantum calculations, we have demonstrated that the optical response of the ubiquitous Au 144 (SR) 60 cluster compound is characterized by a rich fine structure hitherto unknown in spite of the large number of previous experiments and applications. The implications of our results are manifold. For a compound such as the very stable Au 144 (SR) 60 cluster, which can be produced and isolated with utmost precision and reproducibility, they may open the pathway to sensing applications of far greater selectivity than what is conceivable based solely on the existence, energy and, possibly, width of a single plasmon band. Applications based on such optical dactylography are even more likely to succeed as the detailed nature of the ligands beyond the staple motives has been found to induce but negligible changes in the spectra. However, future applications arising from the information content of the spectra will necessarily be based on the control and, hence, the understanding of the temperature effects. Our results provide the basis for further refined studies that will undoubtedly advance the understanding of the metal clusters. The detailed study of the distinct spectral features will certainly be correlated with structural probes and thus increase the understanding of the clusters’ physics. This will shed light on the role of the ‘staple motifs’ in the ligands and on disorder effects that influence—and plague—experiments. In particular, the newly found spectral features enable the fine-tuned study of temperature effects in the future. Beyond the obvious practical importance for applications, such as optical sensing and labelling, our findings have far-reaching implications for the understanding and the study of noble-metal clusters. As the high information content of the optical spectra reflects the quantum size effects that distinguish the cluster from the bulk material, its study will undoubtedly lead to an improved understanding of the transition from bulk metals to clusters and, in particular, to insights into the modification of bulk dielectric functions under miniaturization and, ultimately, the breakdown of the concept in small clusters. The exploitation of the newly found richness of spectral quantum information will certainly foster the study and understanding of the fundamental physical effects that endow the cluster materials with their exceptional properties. Comment on the choice of representation of the spectral functions The presentation of the spectral functions in this form ( ω −2 σ ( ω ) versus ℏ ω , or photon energy) requires comment [56] , [57] . We offer three reasons for this choice. First, it facilitates the visualization of the entire spectrum, from the IR to the mid-UV ranges. Moreover, it preserves the integrated absorption of the conventionally plotted spectra, σ ( λ ) versus λ . Finally, it preserves the identity (see below) connecting the optical spectrum to the (static) electronic polarizability, α 0 , which is a conventional measure of electronic delocalization and conductivity or metallic character. The electronic polarizability of globular metal clusters is very large, as compared with molecules or semiconductor clusters of the same dimension but is bounded by the cluster volume—that is, where R is the radius of the metallic cluster and δ is a small correction for the ‘spill-out’ of the conduction electron density. The standard relations connecting the (static) electronic polarizability to the optical absorption spectrum may be written as: wherein the integrand is the spectral function shown, for example, in Fig. 1 and Supplementary Fig. 1 . TD-DFT calculations Optical absorption spectra have been calculated by TD-DFT using the real-space code octopus [58] , [59] and the gradient-corrected PBE exchange-correlation potential. Norm-conserving Troullier–Martins pseudopotentials [60] have been used that include the respective 5 d electrons in the valence (11 valence electrons for each Au atom). Relativistic effects are included as scalar relativistic correction in the radial part of the pseudopotentials. The spacing of the real-space grid was 0.20 Å. The calculation domain was made up of spheres centred around each atom with a radius of 5 Å. In this way, spectra are well converged up to energies of ~5.5–6.0 eV. After a ground-state calculation, optical absorption spectra are calculated using the time-evolution formalism in the standard way as introduced by Yabana et al. [48] where at t =0 a perturbation is applied. Technically, the wave functions are multiplied by a phase factor e ikz that imposes a coherent velocity field and causes a dipole moment to develop as the system evolves freely [48] . We calculated the response for a perturbation in one direction because the high symmetry makes the response of the cluster isotropic. The absorption spectrum is obtained as the Fourier transform of the time-dependent dipole moment [48] , [59] . The method is illustrated in Supplementary Fig. 4 for a 20-atom Ag tetrahedron. The total energy is used to monitor the stability of the propagation. In our calculations, the time step for the propagation was set to 0.00197, fs. The propagation time was 25 fs, and the propagation was carried out by means of the Approximated Enforced Time-Reversal Symmetry propagator [61] as implemented in the octopus code. The results are equivalent to those obtained using the transition-based Casida formalism [62] , [63] . A comparison of the time evolution results with a transition-based calculation is shown in Supplementary Fig. 5 , a comparison between different exchange-correlation functionals in Supplementary Fig. 6 . We use the atomic coordinates obtained in previous work [20] . Chemicals Hydrogen tetrachloroaurate trihydrate (HAuCl 4 ⋅ 3H 2 O, reagent grade), 1-hexanethiol (98%), tetraoctylammonium bromide (Oct4NBr, 98%) and sodium borohydride (NaBH 4 , 99%) were purchased from Aldrich. Extrapure grade toluene, acetone, methanol, ethanol, acetonitrile and dichloromethane were used. Water was purified using a Millipore Milli-Q system (18.2 MΩ cm). All the chemicals were used as obtained without any further purification. Clusters The Au 144 (SR) 60 clusters were synthesized according to a literature procedure [64] with slight modifications. Typically, 0.70 mmol of Oct 4 NBr and 0.70 mmol of HAuCl 4 ⋅ 3H 2 O were combined in 30 ml of methanol. Vigorous stirring (15 min) results in a solution-colour change from light yellow to bright red, indicating the formation of Oct 4 N + AuBr 4 − . At that point, 3.0 mmol hexanethiol (4.3 equivalents) was added to the solution at room temperature, causing an immediate colour change of the reaction mixture to white. After stirring for 1 h, one adds a chilled aqueous NaBH 4 (7.0 mmol in 12 ml) under vigorous stirring, producing an immediate colour change to a dark-black solution, indicating the formation of various gold nanoparticles, which gradually precipitate from the methanol–water solution, over the following 5 h. Centrifugation and decantation of this solution yields the black precipitates, which were then washed with a copious ethanol to remove reaction byproducts (small-molecule and electrolyte residue, including excess free thiols). The product gold–hexanethiolate clusters were then extracted from the precipitated material into dichloromethane solution. The as-obtained material contains Au 144 (SR) 60 as a major product, R=C 6 H 13 , but also smaller quantities of lower-mass clusters (Au 25 (SR) 18 , Au 67 (SR) 35 and Au 102 (SR) 44 ) as well as larger ones in the 70-kDa mass range. Smaller clusters were removed from powder samples by extraction into acetone. From the remaining (acetone-insoluble) material, the purified Au 144 (SR) 60 clusters were extracted repeatedly into 10:13 acetonitrile/dicloromethane solution. Phenylethane-thiolate-capped Au 144 clusters are a gift from Professor Rongchao Jin, who synthesized them using a procedure published elsewere [64] . Characterization Mass spectra were acquired by the matrix-assisted laser desorption ionization (MALDI) method, using a MALDI-TOF Microflex mass spectrometer (Bruker Daltonics) equipped with a standard UV nitrogen laser (337 nm). The accelerating voltage was held at 15 kV and the spectrum was collected in a linear negative ion mode. A 0.7-mM Au 144 (SR) 60 -enriched dichloromethane solution was mixed with a saturated in dichloromethane solution of trans -2-[3-(4- tert -butylphenyl)-2-methyl-2-propenylidene] malononitrile and then applied to the sample plate and air-dried. The representative mass spectrum obtained ( Fig. 7 ) is free of other clusters, and the deduced mass (35,398 Da) matches closely the calculated mass for the singly charged Au 144 (SC 6 H 13 ) 60 [1−] . 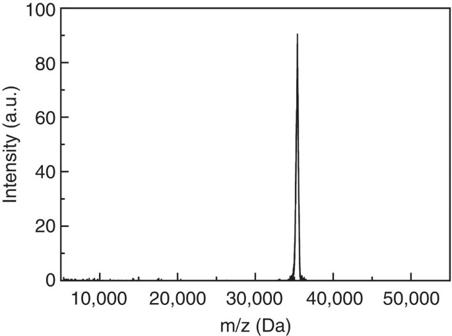Figure 7: MALDI-TOF mass spectrum of Au144(SC6H13)60[1−].  Figure 7: MALDI-TOF mass spectrum of Au 14 4 (SC 6 H 13 ) 60 [1−] . Full size image Optical measurements Ground-state electronic absorption and temperature-dependent absorption measurements were carried out using a CARY-14 UV–vis-NIR absorption spectrophotometer. Au 144 (SC 6 ) 60 clusters were dissolved in methylcyclohexane:methylcyclopentane (1:1) mixture for temperature-dependent absorption measurements as it forms clean glass. An Optistat DN cryostat (Oxford instruments) and an ITC temperature controller were used to carry out the temperature-dependent measurements. The vacuum in the cryostat was maintained with a Leybold turbomolecular pump. The error bars on the temperatures are around 1 K. How to cite this article: Weissker, H.-Ch. et al. Information on quantum states pervades the visible spectrum of the ubiquitous Au 144 (SR) 60 gold nanocluster. Nat. Commun. 5:3785 doi: 10.1038/ncomms4785 (2014).